Identification of a pan-cancer oncogenic microRNA superfamily anchored by a central core seed motif MicroRNAs modulate tumorigenesis through suppression of specific genes. As many tumour types rely on overlapping oncogenic pathways, a core set of microRNAs may exist, which consistently drives or suppresses tumorigenesis in many cancer types. Here we integrate The Cancer Genome Atlas (TCGA) pan-cancer data set with a microRNA target atlas composed of publicly available Argonaute Crosslinking Immunoprecipitation (AGO-CLIP) data to identify pan-tumour microRNA drivers of cancer. Through this analysis, we show a pan-cancer, coregulated oncogenic microRNA ‘superfamily’ consisting of the miR-17, miR-19, miR-130, miR-93, miR-18, miR-455 and miR-210 seed families, which cotargets critical tumour suppressors via a central GUGC core motif. We subsequently define mutations in microRNA target sites using the AGO-CLIP microRNA target atlas and TCGA exome-sequencing data. These combined analyses identify pan-cancer oncogenic cotargeting of the phosphoinositide 3-kinase, TGFβ and p53 pathways by the miR-17-19-130 superfamily members. MicroRNAs are single-stranded RNA molecules ( ∼ 22 nucleotides) that repress messenger RNA translation [1] and promote mRNA degradation [2] , [3] . MicroRNAs are critical regulators of oncogenesis and their regulation of cancer cell signalling is complex. Global microRNA expression is often repressed in cancer [4] , [5] , [6] , [7] . However, some microRNAs are oncogenic [7] , [8] , [9] , [10] , exhibiting amplified expression in many tumour types. Facilitated by Argonaute proteins, microRNAs bind target mRNAs in the RNA-induced silencing complex. MicroRNA target regulation is canonically mediated by nucleotides 2–8 on the 5′-end of the microRNA strand, termed the microRNA seed [11] . A minimum of six consecutive nucleotides is required to pair the microRNA with its target mRNA [11] , [12] . This minimal binding requirement allows a given microRNA to potentially bind tens, hundreds or thousands of mRNA targets [13] . One difficulty in determining the functions of microRNAs in tumours is the wide array of potential genes that any microRNA might regulate. Established microRNA target prediction algorithms are based on inference, relying on evolutionary conservation of 3′-untranslated region (UTR) sequences complementary to the microRNA seed and biochemical binding context to determine putative microRNA binding sites [14] , [15] . Although these algorithms are useful for predicting microRNA targets, especially within the 3′-UTRs, they are not experimental demonstrations of microRNA–target interactions and are often less able to accurately predict microRNA binding within protein-coding regions and non-coding RNAs (ncRNAs) because of reliance on site-specific conservation [11] . Argonaute Crosslinking Immunoprecipitation (AGO-CLIP) data sets experimentally identify microRNA–target interactions in a genome-wide manner through purification of Argonaute-protein-associated RNAs, which include bound microRNAs and their respective targets [16] , [17] , [18] . In this study, to explore the microRNA regulatory landscape across the TCGA Pan-Cancer project [19] , which includes data from breast adenocarcinoma (BRCA), lung adenocarcinoma (LUAD), lung squamous cell carcinoma (LUSC), uterine corpus endometrioid carcinoma, glioblastoma multiforme (GBM), head and neck squamous cell carcinoma (HNSC), colon and rectal carcinoma (COAD, READ), bladder urothelial carcinoma (BLCA), kidney renal clear cell carcinoma (KIRC), ovarian serous cystadenocarcinoma (OV), uterine corpus endometrial carcinoma (UCEC), and acute myeloid leukemia (LAML), we compiled all publicly available human AGO-CLIP data [17] , [18] , [20] , [21] , [22] , [23] , [24] into a single unified atlas and ranked individual microRNA target sites by total occurrences across data sets. We integrated this substantial atlas of microRNA target sites with TCGA pan-cancer microRNA, mRNA, copy number variation (CNV) and exome-sequencing data sets to discover common microRNA regulatory architecture across tumour types. Finally, we developed an algorithm, miSNP, to infer somatic mutations in these regulatory binding sites. Our analysis represents integration of a new resource, the AGO-CLIP atlas, and TCGA data, creating a method by which we were able to understand microRNA regulatory architectures across multiple tumour types. Collectively, this study identified a pan-cancer oncogenic microRNA (oncomiR) network that cotargets multiple potent tumour suppressors (TS) through a common core seed motif. Global microRNA expression patterns in normal and tumour tissue The TCGA pan-cancer data set represents the single largest compilation of microRNA-sequencing data in cancer produced to date. Global analysis of microRNA expression patterns in 4,186 tumours and 334 normal tissue samples revealed the top 30 microRNAs constitute, on average, ∼ 90% of all microRNA expression across heterogeneous normal tissues. The same 30 microRNAs likewise comprise 80–90% of microRNA expression in tumours ( Fig. 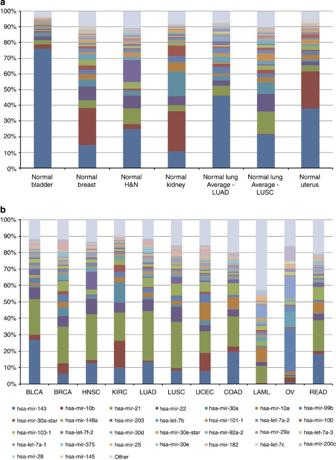Figure 1: The landscape of microRNA expression in the TCGA pan-cancer data set. (a) Thirty microRNAs constitute 90% of microRNA expression across all normal tissues. (b) Global microRNA expression change occurring in tumours is due principally to loss ofmiR-143expression and gain ofmiR-21expression. MicroRNAs represented in columns from bottom to top listed left to right by row legend. 1a,b , Supplementary Tables S1 and S2 ) Figure 1: The landscape of microRNA expression in the TCGA pan-cancer data set. ( a ) Thirty microRNAs constitute 90% of microRNA expression across all normal tissues. ( b ) Global microRNA expression change occurring in tumours is due principally to loss of miR-143 expression and gain of miR-21 expression. MicroRNAs represented in columns from bottom to top listed left to right by row legend. Full size image miR-143 is the single, most highly expressed microRNA in normal tissue, and miR-21 is the most highly expressed microRNA in cancer ( Fig. 1b ). MicroRNA expression patterns undergo global population changes between cancer and normal, primarily due to increased miR-21 expression (from 6.9 to 19% of all microRNA detected) and decreased miR-143 expression (from 33 to 11.2% of detectable microRNA) across tumour types. AGO-CLIP atlas identifies global microRNA binding events AGO-CLIP technology employs ultraviolet crosslinking of RNA to protein followed by immunoprecipitation to determine RNA species bound to the Argonaute protein ( Fig. 2a ). AGO Photoactivatable-Ribonucleoside-Enhanced CLIP (AGO-PAR-CLIP) [17] includes an added step where nucleotide analogues such as 4-thiouridine are introduced before crosslinking. These nucleotide analogues, when crosslinked, undergo T–C transitions during the reverse-transcription step of the AGO-CLIP experiment [17] , allowing more confident visualization of RNA–protein interaction ( Fig. 2b ). 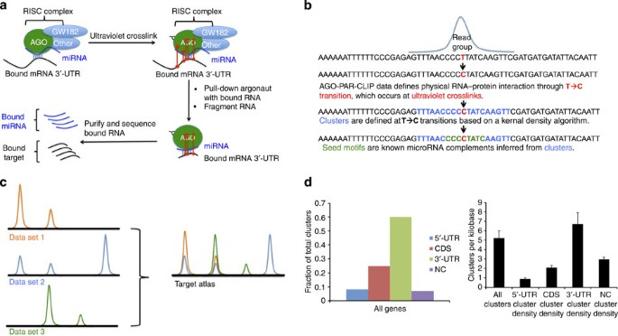Figure 2: Generation of the AGO-CLIP microRNA target atlas. (a) Model of AGO-CLIP-mediated purification of bound microRNAs and target. (b) Example of PAR-CLIP-defined microRNA binding sites.De novoseed identification in this data set requires PAR-CLIP reads. Supplementary identification of recurrent binding sites is allowed for HITS-CLIP data. (c) Construction of seed atlas from multiple data sets emphasizes seeds recurrent across multiple data sets to define high-confidence microRNA active sites. (d) MicroRNA clusters are most frequently mapped to the 3′-UTR region, consistent with previous observations. 3′-UTR, 3′-untranslated region; 5′-UTR, 5′-untranslated region; CDS, coding sequence; NC, non-coding RNA. Error bars represent s.e.m, data is taken from a compilation of 11 AGO-PAR-CLIP libraries used in this study and defined using the 12,449 UCSC known genes with at least one AGO-CLIP cluster mapping to them. Figure 2: Generation of the AGO-CLIP microRNA target atlas. ( a ) Model of AGO-CLIP-mediated purification of bound microRNAs and target. ( b ) Example of PAR-CLIP-defined microRNA binding sites. De novo seed identification in this data set requires PAR-CLIP reads. Supplementary identification of recurrent binding sites is allowed for HITS-CLIP data. ( c ) Construction of seed atlas from multiple data sets emphasizes seeds recurrent across multiple data sets to define high-confidence microRNA active sites. ( d ) MicroRNA clusters are most frequently mapped to the 3′-UTR region, consistent with previous observations. 3′-UTR, 3′-untranslated region; 5′-UTR, 5′-untranslated region; CDS, coding sequence; NC, non-coding RNA. Error bars represent s.e.m, data is taken from a compilation of 11 AGO-PAR-CLIP libraries used in this study and defined using the 12,449 UCSC known genes with at least one AGO-CLIP cluster mapping to them. Full size image We began by generating a large atlas of microRNA binding sites by compiling publicly available AGO-CLIP data ( Supplementary Data 1 ) [17] , [18] , [20] , [21] , [22] , [23] , [24] . This included 11 AGO-PAR-CLIP libraries and 3 unmodified AGO-CLIP libraries (also called Argonaute High-Throughput Sequencing of RNA Isolated by CLIP (AGO-HITS-CLIP)) [16] . The AGO-CLIP atlas allowed us to integrate experimentally defined microRNA–target interactions with TCGA data to create the most accurate prediction of microRNA binding patterns across TCGA cancers. The AGO-CLIP seed atlas consists of 124,000 microRNA target clusters that subsequently infer over 300,000 putative seed motifs within those clusters. Individual seed sites were used as genomic anchors to tabulate recurrent definition of a given seed across 14 AGO-CLIP data sets ( Fig. 2c , Supplementary Data 1 ). Clusters were then randomly permuted across the genome to determine an exact binomial probability of cluster occurrence at a given seed complement. False discovery rates (FDRs) for each seed-complementary target were calculated from their probability of recurrence ( Supplementary Data 1–3 ). We found that ≥3 occurrences of an AGO-CLIP peak on a given target site corresponded to a significant event relative to a random distribution of clusters ( q <0.05 based on binomial P -value, Supplementary Data 3 ). AGO-CLIP defined that cluster localization by mRNA region is largely consistent with previous reports [16] , [17] , with 60% of clusters mapping to the 3′-UTR, 24.7% of clusters mapping to the coding region, 8.2% mapping to the 5′-UTR and 7% mapping to ncRNAs ( Fig. 2d ). DICER1 , MDM2 and the long ncRNA (lncRNA) Xist are among the top ten, most frequently targeted genes in the atlas, suggesting that the microRNA functional roles may include autoregulation, apoptotic sensitization through TP53 and lncRNA function ( Supplementary Data 2 ). Importantly, traditional target prediction algorithms do not predict the high-frequency interactions on both MDM2 and Xist , demonstrating the strength of the unbiased AGO-CLIP platform. We also found numerous interactions between the Argonaute proteins and lncRNAs, small nucleolar RNAs and transfer RNAs in the AGO-CLIP atlas. These findings are consistent with recent evidence, suggesting that ncRNAs are microRNA targets or Argonaute binding substrates [25] . Discovery of these interactions supports a growing consensus that microRNA function extends beyond the regulation of protein-coding genes. Analysis of TCGA microRNA expression data To define which microRNAs consistently change relative to matched normal tissue, we performed significance testing on tumour versus normal microRNA expression levels across samples. Inspection of the TCGA microRNA data set revealed that significance testing (Fisher’s exact test) between tumour and normal samples on the raw reads per million values generated by high-level processed TCGA data produced significantly more increased microRNAs than decreased microRNAs ( Supplementary Fig. S1A ). The reason for this differential significance level between increased and decreased microRNAs is due to loss of highly expressed microRNAs in tumour samples, especially loss of miR-143 , which accounts for 35–70% of microRNA expression in normal tissue. miR-143 expression often decreases by >50% in tumours ( Fig. 1b ). As microRNA expression in sequenced samples is expressed as a population value (reads per million microRNAs mapped), and because total RNA between tumour and normal samples used in sequencing experiments is constant, the loss of miR-143 leads to reciprocal gains in the proportion of other microRNAs. This relationship is demonstrated by the strong association of the absolute number of significantly increased microRNAs and the loss of miR-143 ( R 2 =−0.86, P =0.01, Supplementary Fig. S1B ). We corrected for these composition differences using upper quartile and trimmed median of M -values to normalize the data set [26] . These methods are designed to compensate for differences between tissues (for example, comparing the liver and the kidney) and are thus useful when comparing tumour versus normal tissue microRNA values, because they compensate for artefact generated by large expression changes in the most prevalent microRNAs ( Supplementary Fig. S1A–D ; Supplementary Data 4 contains detailed significance calculations for microRNAs in all tumour types). Definition of microRNA–target interactions We next defined pan-cancer oncomiRs and miR suppressors (tumour-suppressing microRNAs) based on consistent expression changes across cancer types. Pan-cancer oncomiRs were defined by significant expression gain ( q <0.05, Fisher’s exact test) in at least six out of seven pan-cancer tumour types containing tumour versus normal microRNA-sequencing data. Pan-cancer miR suppressors were similarly defined by significant expression loss in at least six of seven tumour types ( Fig. 3a ; Supplementary Data 5 contains detailed pan-cancer microRNA selection data). To ensure we were observing target interactions with highly expressed microRNAs that had many conserved target sites in the 3′-UTR, we focused on the dominant arms of the 87 broadly conserved microRNA families with an Argonaute-bound read group corresponding to the microRNA in at least 3 of the 14 AGO-CLIP data sets in our analysis. 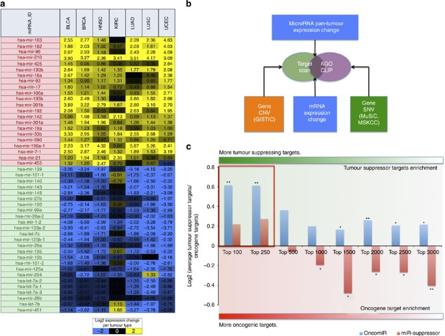Figure 3: Determination of pan-cancer microRNAs and their targets. (a) List of broadly conserved pan-cancer oncomiRs and miR suppressors reveals microRNAs undergoing consistent expression changes across the pan-cancer data set. (b) A dual nomination strategy uses AGO-CLIP microRNA target definitions to associate pan-cancer microRNAs to respective TS and OC targets to define relevant pan-tumour microRNA–target relationships. (c) TS target versus oncomiR target enrichments for pan-cancer oncomiRs (blue bars) and miR suppressors (red bars) across the top 100–3,000 (∼10% of genes) TS and OCs. This graph represents the enrichments and significance levels of those enrichments of both pan-cancer oncomiRs and miR suppressors. Individual bars in the graph represent the log2-based per cent TS over per cent OC targets. Positive bars demonstrate average total enrichment for TS. Negative bars demonstrate average enrichment for OCs. An asterisk defines significant enrichments. Red box highlights enrichment of pan-cancer oncomiRs with their top 250 targets used in subsequent analysis. Student’st-test, *P<0.05, **P<0.005.N-values for enrichment reflect the total number of pan-cancer oncomiRs (n=22) and pan-cancer miR suppressors (n=25). Figure 3: Determination of pan-cancer microRNAs and their targets. ( a ) List of broadly conserved pan-cancer oncomiRs and miR suppressors reveals microRNAs undergoing consistent expression changes across the pan-cancer data set. ( b ) A dual nomination strategy uses AGO-CLIP microRNA target definitions to associate pan-cancer microRNAs to respective TS and OC targets to define relevant pan-tumour microRNA–target relationships. ( c ) TS target versus oncomiR target enrichments for pan-cancer oncomiRs (blue bars) and miR suppressors (red bars) across the top 100–3,000 ( ∼ 10% of genes) TS and OCs. This graph represents the enrichments and significance levels of those enrichments of both pan-cancer oncomiRs and miR suppressors. Individual bars in the graph represent the log2-based per cent TS over per cent OC targets. Positive bars demonstrate average total enrichment for TS. Negative bars demonstrate average enrichment for OCs. An asterisk defines significant enrichments. Red box highlights enrichment of pan-cancer oncomiRs with their top 250 targets used in subsequent analysis. Student’s t -test, * P <0.05, ** P <0.005. N -values for enrichment reflect the total number of pan-cancer oncomiRs ( n =22) and pan-cancer miR suppressors ( n =25). Full size image We examined interactions between putative pan-cancer oncomiRs or miR suppressors, and their driver targets, based on the assumption that pan-cancer oncomiRs are enriched for TS targets and pan-cancer miR suppressors are enriched for oncogenic targets. We then performed integrative analysis of pan-cancer TS and oncogenes (OCs) by using available pan-cancer data, including exome-sequencing single-nucleotide variation (SNV) scores (MuSiC [27] , [28] and MSKCC [29] algorithms), CNV analysis (GISTIC [30] , [31] algorithm) and mRNA expression changes as building blocks for integrated gene nomination ( Fig. 3b ). We generated a continuous scale of relevant pan-cancer genes that describes putative TS as increasingly negative values and putative OCs as increasingly positive values, based on SNV, CNV and mRNA expression changes across TCGA tumour types ( Supplementary Data 6 and Methods). We tested four methods for calling microRNA–target interactions including the following: using all AGO-CLIP-defined binding sites without considering site conservation (for example, TargetScan); using only AGO-CLIP-defined sites with ≥3 occurrences (corresponding to a significant peak based on random permutation) without considering TargetScan; using TargetScan-only binding sites (without considering AGO-CLIP data); and, finally, combining AGO-CLIP-defined target sites with ≥3 occurrences, or ≥1 occurrences and a TargetScan call. We found that combining AGO-CLIP and TargetScan results (final method) was the only method that produced enrichments of TS targets for pan-cancer oncomiRs and OC targets for pan-cancer miR suppressors ( Fig. 3c , Supplementary Fig. S2A–D ). To gain insight into the differing enrichments, we explored the target spectrums of AGO-CLIP-defined target sites and TargetScan-defined target sites for the selected pan-cancer microRNAs. We found that on average 25.6% of TargetScan targets are also nominated by AGO-CLIP. Reciprocally, Target-Scan also nominates 31.47% of AGO-CLIP targets. In total, 74.4% of all TargetScan targets were not called by AGO-CLIP, and TargetScan did not call 68.53% of AGO-CLIP targets. In the case of AGO-CLIP, 34.61% of all targets were outside the 3′-UTR (coding region or 5′-UTR), leaving another 34.39% of all AGO-CLIP-defined targets within the 3′-UTR but not called by TargetScan (results are summarized in Supplementary Table S3 ). Calling interactions using the AGO-CLIP atlas alone produced bias towards enrichment of OCs ( Supplementary Fig. S2A,B ), whereas TargetScan alone produced bias towards TS ( Supplementary Fig. S2C ). The AGO-CLIP data set produces slight bias towards OCs, because the top 3,000 OCs have 31% more AGO-CLIP clusters binding them than the top 3,000 TS. This observation may reflect overexpression of these OCs in the cell lines used to perform the AGO-CLIP analyses, or it may reflect greater microRNA binding of OCs in general, which is consistent with the tumour-suppressive function of many microRNAs [4] , [5] , [6] , [7] . Notably, most of the targeting discrepancy between TS and OCs is due to microRNA binding in the coding region, with OCs having 66% more AGO-CLIP clusters than TS ( Supplementary Fig. S3A ). TargetScan cannot predict microRNA binding in coding regions of genes. TargetScan may produce bias towards TS, because the top 3,000 TS have 40% larger 3′-UTR lengths than the top 3,000 OCs ( Supplementary Fig. S3B ). The relative size of the 3′-UTR directly determines the total number of predicted microRNA target sites associated with that 3′-UTR, suggesting that TS undergo greater 3′-UTR-mediated cis -regulation in general. As many cell lines are rapidly growing or are oncogenic, the relative lack of AGO-CLIP clusters on the TS may reflect the cellular context of the AGO-CLIP experiments wherein these genes could have reduced expression owing to culturing conditions, rather than representing a general phenomenon. Ultimately, determining microRNA–target interactions using AGO-CLIP-defined target sites with ≥3 occurrences, or ≥1 occurrences, and a TargetScan call was the only method to generate expected enrichments in TS targets for oncomiRs and OC targets for miR suppressors. This method had the added utility of combining target site conservation with genomic experimental validation. Discovering expected enrichments when combining TargetScan and AGO-CLIP values may suggest that combined microRNA target calling yields improved accuracy over a single method by reducing the false negatives and false positives inherent in each technology. As such, we chose to define a microRNA–target interaction as ≥3 AGO-CLIP-defined occurrences, or ≥1 occurrences, and a TargetScan for subsequent analysis of tumour-driving microRNA–target interactions. Identification of a pan-cancer oncomiR network We observed that the strongest overall microRNA–target enrichment was for oncomiRs targeting the top 250 ranking TS ( Fig. 3c , red box). Many of these interactions involved cotargeting of multiple microRNAs on the same TS. As many top TS targets were cotargeted by the pan-cancer oncomiRs, we analysed seed sequences of pan-cancer oncomiRs to determine whether any core sequences were common to the individual oncomiR seeds. Intriguingly, 10 of 22 (45.4%, Fig. 4a ) pan-cancer oncomiRs in our analysis share similar sequence homology in their seed region that aligns around a central GUGC motif defining a microRNA seed ‘superfamily’. GUGC motifs occur in 36 of 187 (ref. 13 ) microRNAs from broadly conserved seed families (5.19%), enriching seed families with a GUGC motif in their seed region 8.7-fold among pan-cancer oncomiRs compared with all broadly conserved microRNAs ( P =0.008, Wilcoxon rank-sum test, Fig. 4a ). None of the 25 pan-tumour miR suppressors identified in our analysis contain a GUGC motif, making this motif significantly depleted among the identified miR suppressors ( P =0.016, Wilcoxon rank-sum test). This motif is also enriched when including all microRNAs meeting our significance threshold, and not just the microRNAs from broadly conserved families ( P =5E−10, Wilcoxon rank-sum test; the GUGC motif is present in 4.6% of all dominant-arm miRbase microRNAs and 26% of all microRNAs significantly increased in 6/7 TCGA tumours). 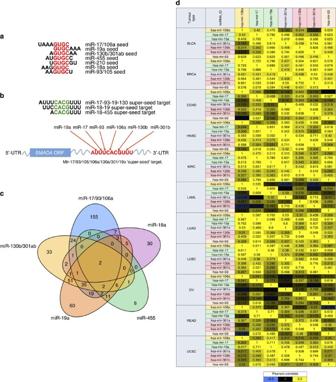Figure 4: Pan-cancer oncomiRs are grouped into a coregulated superfamily of pan-oncomiRs. (a) Broadly conserved pan-cancer oncomiRs (45.4%) share a central GUGC seed sequence homology, grouping them into a larger oncomiR ‘superfamily’ consisting of miR-17, -19, -130, -210, -18 and -455 seeds. (b) MicroRNA superfamilies often target complementary ‘super seeds’. (c) Overview of target predictions for the top 3,000 highest-ranked TS for miR-17, -19, -130, -210 -18 and -455 families demonstrates TS cotargeting relationships with 39.2% ofmiR-17/106a/93targets, 70.2% of miR-19 targets, 79.3% ofmiR-130/301abtargets, 42.3.0% ofmiR-18atargets, 75.7%miR-455targets and 62.5% ofmiR-210targets having predicted cotargeting with at least one other superfamily member. ThemiR-93family has largely the same predicted target spectrum as that of themiR-17family.miR-210has few AGO-CLIP-defined targets and was thus not included in the Venn.miR-93is grouped with themiR-17family in this analysis, because their target spectrums almost completely overlap. The microRNA-17, -19 and -130 families most heavily mediate pan-cancer cotargeting. (d) miR-17-19-130 superfamily members are strongly correlated across pan-cancer tumours, demonstrating potent coregulation of these microRNAs (P<1E-200, Student’st-test). MicroRNAs are colour-coded based on co-localization to the same genomic cluster. microRNA–microRNA correlaten-values are as follows: BLCA=95, BRCA=794, COAD=177, HNSC=301, KIRC=466, LAML=173, LUAD=313, LUSC=193, ovarian carcinoma (OV)=225, READ=65 and uterine corpus endometrioid carcinoma (UCEC)=320. Figure 4: Pan-cancer oncomiRs are grouped into a coregulated superfamily of pan-oncomiRs. ( a ) Broadly conserved pan-cancer oncomiRs (45.4%) share a central GUGC seed sequence homology, grouping them into a larger oncomiR ‘superfamily’ consisting of miR-17, -19, -130, -210, -18 and -455 seeds. ( b ) MicroRNA superfamilies often target complementary ‘super seeds’. ( c ) Overview of target predictions for the top 3,000 highest-ranked TS for miR-17, -19, -130, -210 -18 and -455 families demonstrates TS cotargeting relationships with 39.2% of miR-17/106a/93 targets, 70.2% of miR-19 targets, 79.3% of miR-130/301ab targets, 42.3.0% of miR-18a targets, 75.7% miR-455 targets and 62.5% of miR-210 targets having predicted cotargeting with at least one other superfamily member. The miR-93 family has largely the same predicted target spectrum as that of the miR-17 family. miR-210 has few AGO-CLIP-defined targets and was thus not included in the Venn. miR-93 is grouped with the miR-17 family in this analysis, because their target spectrums almost completely overlap. The microRNA-17, -19 and -130 families most heavily mediate pan-cancer cotargeting. ( d ) miR-17-19-130 superfamily members are strongly correlated across pan-cancer tumours, demonstrating potent coregulation of these microRNAs ( P <1E-200, Student’s t -test). MicroRNAs are colour-coded based on co-localization to the same genomic cluster. microRNA–microRNA correlate n -values are as follows: BLCA=95, BRCA=794, COAD=177, HNSC=301, KIRC=466, LAML=173, LUAD=313, LUSC=193, ovarian carcinoma (OV)=225, READ=65 and uterine corpus endometrioid carcinoma (UCEC)=320. Full size image Several superfamily microRNAs ( miR-17/106a , miR-210 , miR-130b/301ab and miR-93/105 ) derive from the same seed family ( Fig. 4a ). The miR-93/105 and miR-17/106a seed families have virtually the same seeds, leading to highly similar predicted target spectrums. miR-17 , miR-106a , miR-18a and miR-19a are part of the well-described miR-17 ∼ 92 oncogenic cluster, also known as oncomiR-1 (refs 9 , 10 , 32 ). MicroRNA seed similarity in the pan-cancer oncomiRs led us to hypothesize that these microRNAs may undergo coordinate regulation to mutually cotarget and suppress critical TS. To test this hypothesis, we defined the target spectrum of the pan-cancer microRNA superfamily ( Fig. 4b,c ). We observed oncogenic microRNA superfamily cotargeting of high-ranking pan-cancer TS such as SMAD4, ZBTB4 and TGFBR2 , often at a single complementary seed-target site we termed a microRNA ‘super-seed’ target, where multiple families of microRNAs bind and regulate a specific 3′-UTR ( Fig. 4b ). In most superfamily oncomiRs, the majority of targets predicted in the top 3,000 TS are shared with at least one other superfamily member, including 70.2% of miR-19 targets, 79.3% of miR-130/301ab targets, 39.2% of miR-17/106a/93 targets, 42.3% of miR-18a targets, 75.7% miR-455 targets and 62.5% of miR-210 targets ( Fig. 4c ). The entire miR-17-19-130-93-455-18-210 superfamily of pan-tumour oncomiRs identified in this analysis forms three separate super-seed target sites; one consisting of the miR-17, miR-19 and miR-130 families, one consisting of the miR-18 and miR-19 families, and one consisting of the miR-19 and miR-455 families ( Fig. 4b ). The miR-17, miR-19 and miR-130 seed families exhibited the majority of total TS cotargeting on high-ranking TS in our data set. We thus focused further studies on tumour regulation by this subset of oncomiRs. To test possible coregulation of the miR-17, miR-19 and miR-130 families, we correlated the expression levels of family members across TCGA tumours and found strong positive correlation of these microRNAs (average miR-17-19-130 family member microRNA–microRNA correlate across 11 tumour types, R 2 =0.33, P <1E−200 versus null distribution, Student’s t -test, Fig. 4d ). These data suggest that the miR-17-19-130 superfamily members undergo coordinate regulation in tumours to mediate silencing of TS genes in a synergistic manner. To demonstrate the potential for cotargeting of TS by the miR-17-19-130 superfamily members, we determined pan-cancer correlates for all microRNA–target interactions in the top 250-ranked TS. Pan-cancer correlation of high-ranking TS targeted by the miR-17-19-130 superfamily revealed strong negative correlation of the superfamily with many pan-cancer TS, including PTEN , ZBTB4 and TGFBR2 , across all tumour types. 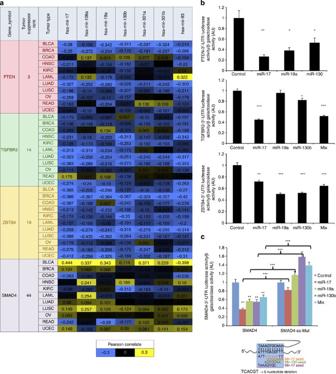Figure 5: The miR-17-19-130 pan-cancer oncomiR superfamily binds and suppresses potent pan-cancer suppressor genes. (a) miR-17-19-130 microRNA–mRNA target correlations across tumours reveals strong negative correlation between superfamily members and their top ranked TS targetsTGFBR2, PTENandZBTB4, but notSMAD4. (b) The miR-17-19-130 superfamily is able to coordinately bind and suppress expression of TS 3′-UTR–luciferase reporter constructs, indicating powerful interaction potential. (c) Superfamily cotargeting on theSMAD43′-UTR occurs at a novel microRNA super-seed locus where multiple microRNA seed families can bind, allowing for potential binding of more than individual microRNAs. Mix, an equimolar mixture of miR-17, -19a and -130b to demonstrate the co-repressive capacity of the oncomiR superfamily as it would exist in the cellular context. *P<0.05, **P<0.005, ***P<0.0005, Student’st-test. Luciferase assays were performed twice at 5 nM mimic and twice at 10 nM in quadruplicate. Results were combined for final analysis (n=16). Error bars are s.e.m. microRNA–mRNA correlaten-values are as follows: BLCA=95, BRCA=794, COAD=177, HNSC=301, KIRC=466, LAML=173, LUAD=313, LUSC=193, ovarian carcinoma (OV)=225, READ=65 and uterine corpus endometrioid carcinoma (UCEC)=320. These numbers reflect the total number of TCGA tumour samples that are characterized with both mRNA and microRNA sequencing. Figure 5a demonstrates correlations with the top four highest-ranked TS ( PTEN , TGFBR2 , ZBTB4 and SMAD4 ) that are targeted by all three seed families. PTEN , TGFBR2 and ZBTB4 , all significantly negatively correlated with the miR-17-19-130 family members versus a null distribution of random microRNA–mRNA correlates ( P <1E−15 for each, Student’s t -test). SMAD4 positively correlates with the superfamily in BLCA ( P <1E−10, Student’s t -test), but otherwise shows no significant correlation, potentially suggesting a role for the microRNAs in translational repression of this target. Full correlate heat map for the microRNA–target pairs in the top 250 TS versus all pan-cancer oncomiRs is provided in Supplementary Data 7 , a complementary heat map for targets of pan-cancer miR suppressors paired with the top 250 OCs is contained in Supplementary Data 8 . Figure 5: The miR-17-19-130 pan-cancer oncomiR superfamily binds and suppresses potent pan-cancer suppressor genes. ( a ) miR-17-19-130 microRNA–mRNA target correlations across tumours reveals strong negative correlation between superfamily members and their top ranked TS targets TGFBR2, PTEN and ZBTB4 , but not SMAD4 . ( b ) The miR-17-19-130 superfamily is able to coordinately bind and suppress expression of TS 3′-UTR–luciferase reporter constructs, indicating powerful interaction potential. ( c ) Superfamily cotargeting on the SMAD4 3′-UTR occurs at a novel microRNA super-seed locus where multiple microRNA seed families can bind, allowing for potential binding of more than individual microRNAs. Mix, an equimolar mixture of miR-17, -19a and -130b to demonstrate the co-repressive capacity of the oncomiR superfamily as it would exist in the cellular context. * P <0.05, ** P <0.005, *** P <0.0005, Student’s t -test. Luciferase assays were performed twice at 5 nM mimic and twice at 10 nM in quadruplicate. Results were combined for final analysis ( n =16). Error bars are s.e.m. microRNA–mRNA correlate n -values are as follows: BLCA=95, BRCA=794, COAD=177, HNSC=301, KIRC=466, LAML=173, LUAD=313, LUSC=193, ovarian carcinoma (OV)=225, READ=65 and uterine corpus endometrioid carcinoma (UCEC)=320. These numbers reflect the total number of TCGA tumour samples that are characterized with both mRNA and microRNA sequencing. Full size image Next, we determined the ability of the miR-17-19-130 family to suppress translation of the top cotargeted TS, PTEN , ZBTB4 , TGFBR2 and SMAD4 using 3′-UTR–luciferase fusions. We used miR-17 , -19a and -130b as representative members of each seed family. We found cosuppressive capacity by pan-cancer oncomiRs on all four pan-cancer TS ( Fig. 5b,c ). In the case of ZBTB4 , PTEN and SMAD4 , all miR-17-19-130 superfamily members were able to bind to the 3′-UTR and significantly repress luciferase activity. miR-19a did not significantly suppress the TGFBR2 3′-UTR ( Fig. 5b ). The SMAD4 gene contains a single miR-17-19-130 super-seed site that is highly conserved and few potential compensatory sites able to bind the miR-17, -19 or -130 seeds. As such, we deleted the central six nucleotides of the SMAD4 super-seed and measured strong ablation of each microRNA seed family’s ability to bind and regulate the SMAD4 3′-UTR ( Fig. 5c ). This finding illustrates the ability of a single 3′-UTR binding site to undergo coregulation by multiple microRNA families at a microRNA ‘super-seed’ target site. 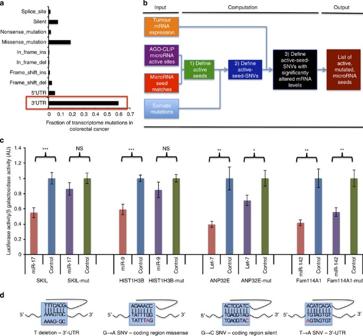Figure 6: The miSNP algorithm defines mutations in microRNA seeds. (a) 3′-UTR mutations make a disproportionate number of all mutations effecting mRNAs. (b) Work flow of miSNP algorithm, which integrates TCGA mutation and mRNA expression analysis and AGO-CLIP seed nominations to determine mutations in active microRNA seeds. (c) Validation of selected AGO-CLIP-defined seed SNVs demonstrates the ability for endogenous tumour mutations to ablate microRNA regulation in a predictable, seed-dependent manner. (d) Mutations reproduced in each 3′UTR construct matching endogenous somatic mutations found in the TCGA pan-cancer data as they relate to the cognate microRNA seed. *P<0.05, **P<0.005, NS, not significant; values measured with Student’st-test. Assays were performed twice at 5 nM mimic and twice at 10 nM in quadruplicate. Results were combined for final analysis (n=16). Error bars are s.e.m. Figure 6: The miSNP algorithm defines mutations in microRNA seeds. ( a ) 3′-UTR mutations make a disproportionate number of all mutations effecting mRNAs. ( b ) Work flow of miSNP algorithm, which integrates TCGA mutation and mRNA expression analysis and AGO-CLIP seed nominations to determine mutations in active microRNA seeds. ( c ) Validation of selected AGO-CLIP-defined seed SNVs demonstrates the ability for endogenous tumour mutations to ablate microRNA regulation in a predictable, seed-dependent manner. ( d ) Mutations reproduced in each 3′UTR construct matching endogenous somatic mutations found in the TCGA pan-cancer data as they relate to the cognate microRNA seed. * P <0.05, ** P <0.005, NS, not significant; values measured with Student’s t -test. Assays were performed twice at 5 nM mimic and twice at 10 nM in quadruplicate. Results were combined for final analysis ( n =16). Error bars are s.e.m. Full size image PTEN is a conserved TS that regulates the oncogenic phosphoinositide 3-kinase pathway [33] . TGFBR2 and SMAD4 are tumour-suppressive components of the transforming growth factor-β (TGFβ) pathway [34] . ZBTB4 is described as a mediator of the p53 response [35] . Thus, the sum of this analysis suggests that the pan-cancer oncomiR superfamily consisting of miR-17, miR-19 and miR-130 seed families coordinately target multiple critical tumour-suppressing pathways across tumour types (modelled in Fig. 7 ). We focused our analysis on the highest-ranking TS targets defined in an unbiased pan-cancer analysis of microRNA–target interactions in this study. Many of the described interactions have been defined previously [9] , [36] , [37] , [38] . However, this study defines these pathway targets as significant across multiple tumour contexts, based on an unbiased estimation of microRNA–target interactions in the largest single data set of human tumours produced to date. Hundreds of potential, novel interactions between these microRNAs and other targets are defined in Supplementary Data 7 . 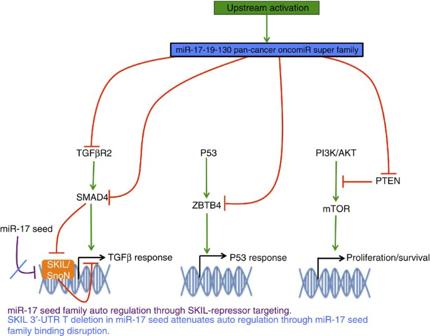Figure 7: A model of Pan-cancer suppressor pathway regulation by miR-17-19-130 superfamily as defined by AGO-CLIP analysis. The microRNA-17-19-130 superfamily heavily targets critical TS in multiple pathways, including the TGFβ pathway, the phosphoinositide 3-kinase/AKT pathway and the P53 pathway. Additional target site mutation analysis reveals ablation of amiR-17-mediated negative feedback loop through mutation of themiR-17binding site on theSKILOC 3′-UTR, demonstrating a novel mechanism of tumour escape from microRNA regulation. Figure 7: A model of Pan-cancer suppressor pathway regulation by miR-17-19-130 superfamily as defined by AGO-CLIP analysis. The microRNA-17-19-130 superfamily heavily targets critical TS in multiple pathways, including the TGFβ pathway, the phosphoinositide 3-kinase/AKT pathway and the P53 pathway. Additional target site mutation analysis reveals ablation of a miR-17 -mediated negative feedback loop through mutation of the miR-17 binding site on the SKIL OC 3′-UTR, demonstrating a novel mechanism of tumour escape from microRNA regulation. Full size image The AGO-CLIP atlas reveals mutations in microRNA targets To define additional novel mechanisms of microRNA regulation in tumours, we next integrated the AGO-CLIP data set with TCGA mutation data to identify somatic SNVs in microRNA target sites across tumours. SNV analysis commonly involves identification of relevant coding-region somatic mutations through predicted functional impacts of amino acid changes associated with the nucleotide variations [27] , [39] . This process, however, remains imperfect. Many missense mutations are not characterized as contributing significant functional impact on a gene. Further, large percentages of coding region mutations are silent. Finally, the number of mutations outside the coding region of genes in regulatory regions (5′-UTR and 3′-UTR) outnumbers coding-region mutations. In our analysis of COAD whole-genome sequencing (WGS) samples, 60% of mutations in coding mRNAs are in the 3′-UTR, highlighting the potential importance of mutations in these regions ( Fig. 6a ). As disruption of microRNA target sites complementary to the microRNA seed region directly interferes with microRNA binding [40] , any mutation in the microRNA target site complementary to the microRNA’s seed is likely to attenuate microRNA control of that site. As such, analysing mutations intersecting with microRNA seed-complementary sites has the potential to greatly expand the search for relevant cancer mutations by imbuing silent mutations and 3′-UTR mutations with functional significance. To perform microRNA seed-target mutation analysis, we developed the miSNP algorithm to integrate AGO-CLIP data with TCGA-defined cancer mutations. miSNP intersects microRNA seed targets with mutation data and retrieves mRNA expression changes corresponding to mutations in these active sites ( Fig. 6b ), providing a powerful method to examine interactions between features and search for subsequent changes in mRNA associated with the interaction. Using the miSNP algorithm, we defined thousands of putative microRNA target-site mutations ( Supplementary Data 9 ). The majority of TCGA pan-cancer SNV data derives from exome sequencing focused solely on coding-region sites. Therefore, the majority of microRNA target mutations we define from the 12 pan-cancer tumours occur specifically in the coding region. Importantly, it is only because we utilize the AGO-CLIP technology that we are able to define these microRNA target-site mutations at all. In addition, KIRC exome sequencing has a small number of 3′-UTR mutations annotated and we incorporated 36 COAD WGS samples that contain full 3′-UTR SNV annotations. To demonstrate the ability of the AGO-CLIP technology and the miSNP algorithm to detect relevant microRNA target-site mutations, we selected six binding site mutations for experimental validation ( Supplementary Data 10 ). These sites were chosen based on the number of times the specific binding site was identified in the AGO-CLIP atlas, the location of the seed in the coding region or 3′-UTR, whether TargetScan called the site as highly conserved and the relative location of the mutation within the seed-complementary region of the binding site. This selection included three mutations in 3′-UTR sequences and three mutations in coding sequences to capture the diversity of the miSNP analysis ( Supplementary Data 10 ). Four of six tested microRNA binding sites with corresponding somatic mutations demonstrated strong evidence of microRNA binding and regulation of the selected site, silencing luciferase expression by >40% in each case and strongly suggesting our analysis identifies functional microRNA binding sites ( Fig. 6c ). For the four target sites with validated target repression, we reproduced the endogenous tumour mutation in the 3′-UTR–luciferase construct. The binding site SNVs corresponding to the miR-17 seed on the SKIL 3′-UTR and the miR-9 seeds on the HIST1H3B 3′-UTR were able to ablate microRNA binding. Mutations complementary to the Let-7 seed on ANP32E and miR-142 seed on FAM114A1 variably reduced, but did not ablate, the repressive ability of the microRNA on the luciferase reporter ( Fig. 6c ). The ability of a mutation to ablate microRNA binding was directly related to the relative position of the mutation within the region complementary to the microRNA seed. Mutations in the first or last nucleotide of the seed complement had a reduced ability to ablate binding relative to mutations near the centre of the seed complement ( Fig. 6d ). These observations are consistent with established concepts of microRNA binding [40] and demonstrate the ability to tier the probable functional impact of microRNA binding site mutations based on its location within the seed-complementary region of the mRNA target. One microRNA target site mutation validated in our study was a deletion of a miR-17 seed family binding site in the SKI-like OC ( SKIL/SnoN ) 3′-UTR. SKIL is a known OC and was ranked in the top 7% of pan-cancer OCs in our pan-cancer mRNA driver index due to expression gain and copy number amplification ( Supplementary Data 6 ). SKIL oncogenic function is known to occur through direct repression of the TGFβ signalling pathway, and part of the TGFβ signalling pathway activation involves targeting and degradation of the SKIL protein [41] , [42] , [43] . Targeting of the SKIL -3′-UTR by the miR-17 seed family reveals potential autoregulatory feedback that can attenuate silencing of the TGFβ pathway by the miR-17-19-130 superfamily. Mutation of the miR-17 seed-family binding site on the SKIL 3′-UTR may represent a mechanism to allow escape from this feedback regulation, allowing unregulated SKIL expression while simultaneously enhancing the oncogenicity of the miR-17 seed family and creating enhanced suppression of the TGFβ pathway ( Fig. 7 ). The miR-17 seed-family binding site on the SKIL 3′-UTR is identified in 8 out of 14 AGO-CLIP data sets, indicating that the site itself is highly active endogenously. Despite this strong evidence of microRNA binding in the AGO-CLIP atlas, TargetScan, Pictar and MiRanda, motif calling algorithms [13] , [14] , [44] , [45] do not nominate SKIL as a potential target of the miR-17 family, again highlighting the value of unbiased genome-wide binding assays as a useful method of determining active microRNA seeds. Combinatorial definition of high-confidence microRNA binding sites using multiple transcriptome-wide AGO-CLIP data sets generated clear evidence of endogenous microRNA binding at specific locations on an mRNA strand. Points of microRNA interaction tested in this study included multiple microRNA binding sites, such as the miR-17-SKIL binding site and binding sites in coding sequences of the mRNA, that are difficult to detect through other means of microRNA target site prediction. We found that 45% of broadly conserved pan-cancer oncomiRs share strong homology in their seed motifs. Seed similarity leads to redundant cotargeting, and therapeutic suppression of any one of these microRNAs is likely to face compensation from other members of the superfamily. The 3′-UTR–luciferase binding assays and anticorrelates of microRNA–target pairs support the possibility that these microRNAs redundantly cotarget important TS across multiple tumour types. The ability of super-seed target sites to bind multiple members of the oncogenic superfamily make them an attractive therapeutic candidate in the future, because it may effectively act as a microRNA ‘sponge’ [46] that can bind and titrate off multiple superfamily members to restore normal cellular regulation in cancer cells by de-repressing critical TS. This therapy may prove more effective than targeting a single oncomiR family, because it has the potential to concurrently sequester multiple oncogenic microRNA seed families to disrupt redundant oncogenic co-repression of TS. Using the miSNP algorithm, we identified thousands of mutations in microRNA binding sites. These mutations were discovered in the exome-sequencing-defined coding-region mutations available from the Pan-Cancer project, a small number of 3′-UTR mutations available from KIRC exome sequencing and whole-genome 3′-UTR mutations from 36 COAD WGS samples. AGO-CLIP characterization of microRNA binding in additional tissue types and integration of additional 3′-UTR mutations from broader cohorts of WGS samples will improve the yield of relevant microRNA target site mutations in the future. In conclusion, we generated a novel resource, the AGO-CLIP atlas, to integrate experimentally defined microRNA binding sites with TCGA tumour data, creating a new method and framework to understand microRNA regulation of cancer. This method addresses the difficult question of determining accurate genome-wide microRNA–target interactions. Integration of the AGO-CLIP-defined microRNA-binding data with TCGA tumour data revealed several novel insights into microRNA regulation of human tumours, including the definition of a pan-cancer oncomiR superfamily and genome-wide identification of microRNA-binding site mutations. Argonaute Crosslinking Immunoprecipitation AGO-CLIP sequence read archive (SRR) files corresponding to all publicly available human AGO-CLIP experiments were downloaded from the NIH sequence read archive (SRR codes: SRR048973, SRR048974, SRR048975, SRR048976, SRR048977, SRR048978, SRR048979, SRR048980, SRR048981, SRR359787, SRR189786, SRR189787, SRR189784, SRR189785, SRR189782, SRR189783, SRR580362, SRR580363, SRR580352, SRR580353, SRR580354, SRR580355, SRR580359, SRR580360, SRR580361, SRR580356, SRR580357, SRR343336, SRR343337, SRR343334, SRR343335, SRR592689, SRR592688, SRR592687, SRR592686, SRR592685; data were downloaded on 11 January 2013). Files were individually pre-processed using Fastx toolkit and cut-adapt to remove adaptor sequences and control for sequence quality. Data set quality was individually discerned using Fast QC reader. Individual sequencing runs were tiered and grouped, based first on group publishing, on cell line used, then on individual treatment and finally based on total reads. In this manner, 14 independent AGO-CLIP data sets were defined (summarized in Supplementary Data 1 ). Individual cell lines with correspondent AGO-CLIP data include: 293T (4/14 experiments), hESC (1/14 experiments), BCBL1 (1/14 experiments), BC-3 (2/14 experiments), BC-1 (1/14 experiments), LCL35 (1/14 experiments), LCL-BAC (1/14 experiments), LCL-BAC-EBV-infected (2/14 experiments) and EF3D (1/14 experiments). Eleven of these data sets were AGO-PAR-CLIP experiments. Three were AGO-HITS-CLIP experiments. Reads from both experiment types were mapped to hg19 using established Bowtie parameters [47] . Both HITS-CLIP and PAR-CLIP methods utilize ultraviolet crosslinking of RNA-binding proteins to their respective RNA partners, followed by protein immunoprecipitation and high-throughput sequencing of the bound RNA. The difference between the two methods lies in the use of photoactivatable ribonucleoside analogues in PAR-CLIP data sets, which allow experimental determination of physical interlinkage between protein–RNA pairs through a mismatch repair defect initialized at crosslinked nucleoside analogues during complementary DNA synthesis, leading to T→C transitions in the generated cDNA. Of the two, the majority of human data sets are PAR-CLIP generated, and an established pipeline exists for processing of these data forms [48] . This pipeline algorithm, termed PARalyzer, uses a kernel-density algorithm centred on crosslinks to generate putative microRNA target sites. In the PARalyzer algorithm, reads are first processed into read groups based on total number of reads. T→C transitions in read groups are then used to define clusters based on the kernel-density algorithm. Cluster sequences then undergo motif analysis for complements of microRNA seeds to infer the identity of the microRNA binding partner. PAR-CLIP Bowtie files were processed through the PARalyzer [47] algorithm to generate clusters and seeds using established parameters [47] . AGO-HITS-CLIP Bowtie files were also processed through PARalyzer and group data were isolated. AGO-HITS-CLIP data groups were superimposed over microRNA target sites identified by the PAR-CLIP reads. In this way, AGO-CLIP data sets were allowed to support the strength of a target site identified in the PAR-CLIP runs by contributing to site recurrence, but were not allowed to perform de novo target site identification. Meta-analyses concerning the location of clusters and their density on various segments of the transcriptome (3′-UTR, coding sequence and 5′-UTR) were performed using only the 11 AGO-PAR-CLIP libraries. A lenient seed inference strategy was used, which included all miRBase seed families. The purpose of this lenient mapping was to anchor redundant read clusters to the genome to determine seed-site recurrence across all data sets. Using this strategy, 99% of 123,752 PAR-CLIP clusters mapping to the UCSC known gene transcriptome received at least one seed inference, although likely to be at the expense of false positives in less-expressed microRNAs. From these cluster sequences, 306,733 microRNA seed-complementary sequences were inferred. Multiple seed complements may be inferred from a single cluster sequence and these seeds often overlap a single site. These sites often highlight putative microRNA super-seed targets, which are readily apparent in AGO-CLIP data. The identity of the actual binding partner may be one of the complementary microRNAs, all of them, or may represent a form of non-canonical binding that is not currently considered in our motif analysis [25] , [48] . Following target identification, the seed complements of each target were grouped for recurrence across the 11 PAR-CLIP data sets. To this, 3 HITS-CLIP read groups were intersected to combine data from 14 total AGO-CLIP sources. PAR-CLIP clusters and HITS-CLIP groups were then permutated across the genome 20 times using BedTools [49] and analysis was performed to determine the likelihood of a given target being recurrently identified by chance after randomization. A FDR was assigned based on binomial P -values established from the actual measured probability of a seed-complementary site recurring at random based on random distribution of the target sites across the transcriptome. We determined target site recurrence of three or more corresponded to a Q -value <0.05. TCGA data acquisition All TCGA data, except for microRNA expression, were downloaded from the Synapse archive as part of the TCGA Pan-Cancer project and correspond to TCGA pan-cancer whitelist files (originally downloaded 25 January 2013). The TCGA Pan-Cancer project consists of 12 available tumour types that include COAD, READ, LUAD, LUSC, BLCA, BRCA, GBM, UCEC, KIRC, LAML, OV and HNSC. Some components of available data are currently incomplete, such as missing normal microRNA-sequencing samples for LAML, ovarian carcinoma, GBM, COAD and READ. MicroRNA data were compiled individually from the TCGA data portal to analyse microRNA isoform data, which were not present on Synapse at the time of analysis. MicroRNA data were processed directly from the TCGA data portal isoform files for all whitelist tumours as of 20 November 2012. Multiple reads from an individual isoform were collapsed into a single read count; the reads per million microRNAs mapped data form was used, which establishes each microRNA read count as a fraction of the total microRNA population. MicroRNA-sequencing data used in this study are summarized in Supplementary Table S1 . MicroRNA data underwent upper-quartile normalization [50] using the edgeR software package [51] , which produced the best overall normalization results compared with reads per million or trimmed median of M -values [52] normalization, followed by determination of significant differences between tumour and normal samples using a Fisher’s exact test with Bonferroni correction to determine FDRs. As part of the Pan-Cancer project, some processed data were available for second-line analysis. These data included pan-cancer CNV data processed through the ABSOLUTE-GISTIC [31] pipeline and mutation data processed through the MuSiC [28] suite and the MSKCC driver analytical pipeline, which were incorporated into driver gene nominations. A list of data IDs in Synapse is provided in Supplementary Table S4 . Pan-cancer oncomiR and miR-suppressor selection Our goal in nominating pan-cancer oncomiRs and miR suppressors was to determine microRNAs that change consistently in the same direction across most cancers. Thus, we set a stringent ( q <0.05, Fisher’s exact test with Bonferroni correction for multiple testing) threshold comparing tumour versus normal microRNA expression, and required pan-cancer oncomiRs to have increased expression in six out of seven tumour types with available tumour versus normal data. Alternately, pan-cancer miR suppressors were required to have decreased expression in six out of seven tumour types. Finally, when determining microRNAs to analyse for microRNA–target interactions, we additionally filtered for dominant isoforms in broadly conserved microRNA families that have peaks identified in at least 3 of 14 AGO-CLIP data sets. This helped limit false positives in the microRNA–target analysis by ensuring the interactions we observed consisted of conserved microRNA seeds derived from microRNAs expressed in the AGO-CLIP cell lines. TS and OC definitions This analysis utilized three external data sets generated for the purpose of pan-cancer analysis by the TCGA: MuSiC, MSKCC driver target analysis and GISTIC. The strength of the MuSiC algorithm, developed at Washington University [25] , is its ability to quality-control SNV samples, eliminate outliers (such as certain hypermutated samples) and derive P -values to determine significantly mutated genes versus the background mutation rate. We thus utilize MuSiC P -values and mutation frequencies in our analysis. Specific mutations are likely to either activate or inactivate genes, and definition of these mutation sites in a single gene can ultimately define that gene as an OC or TS. The MSKCC algorithm [29] creates a binary definition of SNVs that we are able to use to stratify mutated genes as either OCs or TS based on a functional impact score that weighs the probable impact of mutation at a specific amino acid residue. Finally, GISTIC [30] , developed at the Broad Institute, is an algorithm that controls for sample quality and low-amplitude copy number shifts in CNV data derived from single-nucleotide polymorphism arrays. We utilized processed GISTIC data to define CNV log ratios and set CNV thresholds. Our mRNA q -values are performed in house and set at stringent, common threshold value ( q <0.005, Student’s t -test with Bonferroni correction). A ranking system was developed, which integrates TCGA mRNA, CNV and mutation data analysed by TCGA data available from the MuSiC, MSKCC driver target and GISTIC algorithms. This system equally weighted CNV, mRNA expression change and gene mutations as three orthogonal methods of identifying TS and OCs across tumours. This method generated a continuous ranked list for every gene, based on consistent changes across tumours, ranging from more negative (TS) to more positive (OCs). For mRNA data, +1 point was given for each of seven tumours with microRNA-seq data available, in which there was a tumour versus normal significant increase (Student’s t -test, q <0.005), and −1 point was assigned for significant decreases in mRNA expression. For CNV data, GISTIC scores for HUGO-gene-annotated locus copy-number changes were used. We set an amplification/deletion threshold of 0.3 or −0.3 for each sample. For each whitelist tumour in which a given gene achieved amplification or in 30% of samples, +0.5 or −0.5 points was awarded accordingly. Finally, for mutation scores, MSKCC and MuSiC mutation analyses were both integrated. Gene mutations were only considered based on MuSiC-determined Fisher’s combined P -test FDR q <0.005. Mutation frequency was multiplied by 100 and then by 1 or −1, based on MSKCC driver analysis as a TS (*−1) or an OG (*1). Genes nominated as both TS and OG are negated. Truncating mutations based on MSKCC truncation tabulation were assigned additional significance, and the fraction of truncations/total mutations was multiplied by −5 to attribute additional negative value to any gene with high frequency of truncating mutations. All scores were then summed to generate a final pan-cancer TS versus OC score. In sum, this analysis generated a continuous negative-to-positive scale that ranked pan-cancer drivers based on consistent mRNA, CNV or mutation changes across tumours. These three values were scaled to have roughly equal weight to place equal emphasis on the three orthogonal technologies used in the analysis. The scoring equation is described below: There are six tumours with tumour versus normal mRNA (BLCA, BRCA, HNSC, KIRC, LUAD and LUSC). All tumours contain CNV data and mutation data. Mutation frequency must be significant ( q <0.005, Fisher’s exact test) to be considered at all. The MSKCC mutation analysis assigns +1 or −1, based on whether mutations in a given gene activate or inactivate the gene in question. Final score is weighted so that each independent technology contributes equally to overall scoring. Mutation score is highly dominant in several genes such as TP53 with very high mutation frequencies ( ∼ 50% of all tumours). MicroRNA–target enrichment calculations To define an optimal method of determining microRNA–target interactions, we intersected pan-cancer oncomiRs and miR suppressors with pan-cancer TS versus pan-cancer OCs based on four different possible approaches that included the following: using all AGO-CLIP-defined binding sites without considering site conservation (for example, TargetScan), using only AGO-CLIP-defined sites with ≥3 occurrences (corresponding to a significant peak based on random permutation) without considering TargetScan, TargetScan-only binding sites, and finally by combining AGO-CLIP-defined target sites with ≥3 occurrences, or ≥1 occurrences and a TargetScan call ( Supplementary Fig. S2 ). Only well-conserved TargetScan calls were considered in this analysis. To calculate enrichments, the per cent of total targets per microRNA defined as TS as compared with the per cent of total number of targets defined as OCs for all genes in the top 100, 250, 500, 1,000, 1,500, 2,000, 2,500 and 3,000 TS versus OCs (see Supplementary Fig. S2 for all levels of data and Supplementary Data 6 for complete mRNA driver analysis). The average per cent of TS versus OC targets was compared for oncomiRs and miR suppressors using Student’s t -test based on the following equation: For n number of OC or TS ranked in the top 3,000 ( Supplementary Data 6 ), where n =1→3,000; Cotargeting representation was performed with the Venn Diagram package in R. MicroRNA pan-cancer correlations Two sets of correlations were used in this study. The first was microRNA to microRNA correlation for miR-17-19-130 family members identified as pan-cancer oncomiRs. These correlates consist of a simple microRNA-to-microRNA Pearson’s R 2 value. To generate a null distribution, 100 mature, dominant isoform microRNAs were randomly selected and correlated to all randomly selected microRNAs across tumours. MicroRNAs that were not expressed in a given tumour were filtered out of the analysis. This generated a null distribution of random microRNA correlates (average Pearson’s R 2 =0.02, s.d.=0.11) to which the miR-17-19-130 family correlates were compared. Similarly, for microRNA–mRNA targets, 100 random microRNAs were correlated to 200 random genes. This created a null microRNA–mRNA correlation (average Pearson’s R 2 =0.005, s.d.=0.10). To this combined correlations between the miR-17-19-130 pan-cancer microRNAs and the PTEN , TGFBR2 , SMAD4 and ZBTB4 genes were compared to establish P -values. AGO-CLIP SNV intersection We developed the AGO-CLIP SNV intersection (miSNP) algorithm and software package to investigate the effects of microRNAs on tumour samples by integrating exome-sequencing data, AGO PAR-CLIP microRNA/mRNA binding results and RNA-seq gene expression data across multiple TCGA data sets. miSNP performs two types of integration. First, by using only the mutation data and the AGO PAR-CLIP microRNA/mRNA binding sites, miSNP aggregates and reports at gene level both the microRNA binding sites and the mutations. Data collected for a particular gene include the individual microRNAs targeting the gene, as well as the types of mutations in the microRNA binding sites. Next, miSNP incorporates RNA-seq gene expression data to enable a user to carry out a quantitative analysis of the effects of microRNAs and mutations on gene expression across a TCGA data set. The algorithm operates on a gene-by-gene basis. It first partition the tumour samples into those that contain mutations in microRNA binding site; the algorithm can be customized to consider only particular mutation types (for example, coding, silent). Next, it reports the gene expression data for these genes and samples in a tabular format for further analysis. Finally, it identifies genes for which the expression associates with the mutation status in microRNA binding sites by comparing the gene expression distributions of tumour samples with or without common sites using a two tailed Welch’s t -test; miSNP reports both the fold-change and the t -test P -value for each gene. miSNP was developed in Python utilizing the Numpy and Scipy modules. In the current paper, we analysed all AGO-CLIP-defined microRNA target sites for mutations to define a global perspective of possible interactions, but selected sites for validation only from interactions with ≥3 occurrences corresponding to a non-random event. The miSNP software package ( Supplementary Software 1 ) is an open source (Free BSD license) and is available for community download at: www.genboree.org/miSNP . Luciferase assays The PTEN 3′-UTR–luciferase reporter constructs were purchased from Addgene (Cambridge, MA) [26] , [53] . All other constructs were purchased directly from Switchgear Genomics (Palo Alto, CA) and generated using pLightSwitch_3′-UTR vectors. MicroRNA MirVana mimics and negative control mimic were purchased from Ambion (Grand Island, NY). Luciferase assays were performed using the LightSwitch assay kit according to the SwitchGear LightSwitch luciferase assay kit protocols. Reporter plasmids and microRNA mimics were transfected using Lipofectamine 2000 (Life Technologies, Grand Island, NY). Luciferase activity was normalized to β-galactosidase activity. For coding-region constructs, synthetic binding assays were generated by placing the coding region downstream of the luciferase reporter in the UTR. All binding assays were performed in confluent HEK293T cells for 24 h at 5 and 10 nM concentrations microRNA mimic and 40 ng of luciferase and β-galactosidase vector. Experiments were replicated twice at 5 nM and twice at 10 nM experimental concentrations in quadruplicate, and results were combined for final statistical analysis. Insert sequences novel to this study are available in Supplementary Data 11 . HEK293T cells were a kind gift from Dr Weiwen Long. How to cite this article: Hamilton, M. P. et al . Identification of a pan-cancer oncogenic microRNA superfamily anchored by a central core seed motif. Nat. Commun. 4:2730 doi: 10.1038/ncomms3730 (2013).